GPI-anchored proteins do not reside in ordered domains in the live cell plasma membrane The organization of proteins and lipids in the plasma membrane has been the subject of a long-lasting debate. Membrane rafts of higher lipid chain order were proposed to mediate protein interactions, but have thus far not been directly observed. Here we use protein micropatterning combined with single-molecule tracking to put current models to the test: we rearranged lipid-anchored raft proteins (glycosylphosphatidylinositol(GPI)-anchored-mGFP) directly in the live cell plasma membrane and measured the effect on the local membrane environment. Intriguingly, this treatment does neither nucleate the formation of an ordered membrane phase nor result in any enrichment of nanoscopic-ordered domains within the micropatterned regions. In contrast, we find that immobilized mGFP-GPIs behave as inert obstacles to the diffusion of other membrane constituents without influencing their membrane environment over distances beyond their physical size. Our results indicate that phase partitioning is not a fundamental element of protein organization in the plasma membrane. Since Singer and Nicolson [1] proposed their ‘fluid mosaic’ model, it has become clear that lipids and proteins are not just independent components of the plasma membrane but that their arrangement, dynamics and function are interdependent. Organization and interaction of proteins and lipids have been proposed to occur on different time and length scales, from direct molecular interactions to transient association within nanoscopic domains to the optically resolvable phase separation observed in model systems. It is astonishing, however, that very basic functionalities of the plasma membrane have thus far remained enigmatic [2] . One central open question relates to the role of lipids in modulating interactions between membrane proteins. In this paper we address this question, by measuring, how the presence of a membrane protein influences its molecular environment—lipids and other proteins—in the live cell plasma membrane. On the smallest scale, transmembrane proteins are known to bind a shell of annular lipids [3] . However, the area of influence of a protein can extend beyond that: molecular dynamics simulations recently revealed up to 100 lipid molecules co-diffusing with a single protein molecule in a dynamic complex [4] , with substantial effects on lipids at 1- to 2-nm distance from the protein surface. From the overall densities of proteins and lipids in a cell membrane, Niemela et al . [4] proposed that virtually no free bulk lipid molecules exist in a biological membrane, consistent with earlier experimental work [5] . On a larger scale, the multitude of membrane lipids and proteins is thought to have an inherent tendency to organize according to their molecular affinities. A key molecule in this context seems to be cholesterol, which, because of its rigid sterol backbone, disfavours interactions with the more bulky unsaturated lipid species [6] and preferably associates with saturated lipids [7] and certain proteins [8] , [9] . Indeed, the coexistence of phases of different fluidity and acyl chain order—termed liquid-ordered (Lo) and liquid-disordered (Ld)—in model membranes composed of cholesterol, an unsaturated, and a saturated lipid has been studied extensively [10] . By pinning some of the ordered (or disordered) lipids, these phases can be arranged at will: Piehler and colleagues were able to create Lo/Ld phase regions in polymer-supported lipid membranes, which followed the underlying micropatterned structures imposed on the membrane via palmitic or oleic acids as tethering moieties [11] . Along the ame lines, pinning of dioleoyl-phosphatidylethanolamine (distearoyl-phosphatidylethanolamine) via actin fibres nucleated disordered (ordered) phase formation in bilayers of ternary lipid mixtures [12] . From studies on model systems, it was tempting to propose similar phase coexistence also for cell membranes. Indeed, the live cell plasma membrane seems predestined for phase separation as it contains all the necessary ingredients: unsaturated lipids, saturated lipids (sphingolipids as well as glycosylphosphatidylinositol (GPI)-anchored proteins) and cholesterol. Already in 1997, Simons and Ikonen [13] suggested that the well-known detergent-resistant membrane (DRM) fractions may have an analogue in native cell membranes, and termed these putative structures ‘rafts’. A decade later, Lo/Ld phase separation was also demonstrated in giant plasma membrane vesicles (GPMVs) that can be generated from the plasma membrane of cells after specific treatment [14] . Partitioning of proteins and lipids to ordered and disordered phases was often similar to what was expected from studies on DRMs; for example, mGFP (monomeric green fluorescent protein)-GPI is typically not soluble in nonionic detergents and was found to be highly enriched in the Lo phase in GPMVs [15] , [16] . While phase separation on the microscale has not been observed in the live cell plasma membrane, there is an increasing amount of studies indicating that separate lipid phases may be formed on the nanoscale. It is possible that biological membranes are close to a miscibility critical point [17] , [18] , with pronounced phase fluctuations: recent theoretical work suggests that pinning few molecules can trigger the formation of long-lived connected regions in such near-critical membranes [19] , [20] . Experimental evidence for the presence of raft-like platforms in cells includes the coexistence of more and less ordered membrane environments as inferred from Laurdan imaging in live cells [21] , [22] , the observation of lipid-modulated protein–protein or protein–lipid clusters [23] , [24] , [25] , [26] , [27] and transient halts of lipids observed via spot-variation fluorescence correlation spectroscopy (FCS) [28] . In particular, some GPI-anchored proteins form oligomers, which seem to be stabilized by both protein- and lipid-mediated interactions [29] , [30] , [31] . The underlying mechanisms for all these observations, however, are largely unclear; particularly, there are no experiments showing a direct link between the live cell data and fundamental membrane biophysics. In this study, we directly tested whether predictions from membrane biophysics also hold in the native cell membrane. For this, we micropatterned an Lo phase marker—in our case GPI-anchored mGFP (mGFP-GPI)—in the live cell plasma membrane at various surface densities, and measured the influence on fluorescent tracer lipids and proteins by single-molecule microscopy ( Fig. 1 ). We find that, in contrast to the model membrane studies, other Lo phase markers are not attracted by the immobilized mGFP-GPI, and—even at the highest protein density of 10,000 molecules per μm 2 —we do not observe the formation of a connective phase with altered membrane fluidity. Further, we can exclude any co-enrichment of nanoscopic-ordered membrane domains within mGFP-GPI micropatterns. The immobilized mGFP-GPI molecules essentially act as simple obstacles to the movement of other membrane constituents. From the reduction in mobility we determine the reach of the immobilized proteins with respect to the mobile tracers: CD59—another GPI-anchored protein—senses the 2.5-nm diameter of the mGFP β-barrel, whereas Chol-KK114—a fluorescent cholesterol analogue—is able to approach even the 1.6-nm-sized acyl chains of the immobilized mGFP-GPI. 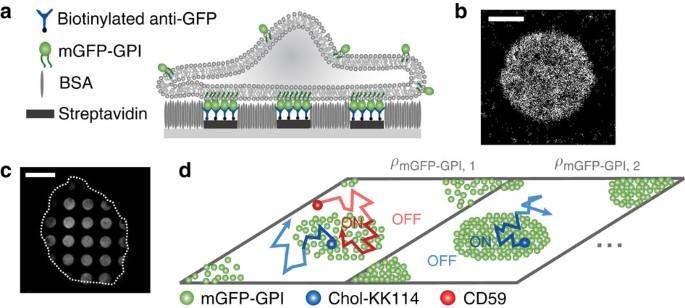Figure 1: mGFP-GPI patterning scheme. (a) Cells stably transfected with mGFP-GPI were grown on micropatterned glass coverslips containing 3-μm-sized spots of GFP antibody; interspaces were passivated by BSA. mGFP-GPI became locally immobilized and enriched at plasma membrane regions coinciding with the GFP antibody patterns. (b) PALM image of psCFP-2 bound to anti-GFP patterns. Scale bar, 1 μm. (c) Total internal reflection fluorescence microscopy (TIRFM) image of a cell grown on micropatterns. mGFP-GPI clearly follows the antibody patterns. The cell outline is indicated by the dashed white contour line. Scale bar, 10 μm. (d) Schematic of our approach. Cells are grown on slides with micropatterns containing different amounts of GFP antibody, so that different surface densities of immobilized mGFP-GPI,ρ, can be adjusted in the plasma membrane. Localizations and mobilities of a probe (CD59 or Chol-KK114) are determined for mGFP-GPI-enriched (ON) and -depleted (OFF) areas. Figure 1: mGFP-GPI patterning scheme. ( a ) Cells stably transfected with mGFP-GPI were grown on micropatterned glass coverslips containing 3-μm-sized spots of GFP antibody; interspaces were passivated by BSA. mGFP-GPI became locally immobilized and enriched at plasma membrane regions coinciding with the GFP antibody patterns. ( b ) PALM image of psCFP-2 bound to anti-GFP patterns. Scale bar, 1 μm. ( c ) Total internal reflection fluorescence microscopy (TIRFM) image of a cell grown on micropatterns. mGFP-GPI clearly follows the antibody patterns. The cell outline is indicated by the dashed white contour line. Scale bar, 10 μm. ( d ) Schematic of our approach. Cells are grown on slides with micropatterns containing different amounts of GFP antibody, so that different surface densities of immobilized mGFP-GPI, ρ , can be adjusted in the plasma membrane. Localizations and mobilities of a probe (CD59 or Chol-KK114) are determined for mGFP-GPI-enriched (ON) and -depleted (OFF) areas. Full size image Immobilizing mGFP-GPI within patterns in the plasma membrane mGFP-GPI is known to preferentially partition into the ordered phase of phase-separated GPMVs [15] , was found in DRM fractions [16] and is typically regarded as a bona fide raft marker. Moreover, it is devoid of any cellular functions and does not show substantial tendencies to associate with other GPI-anchored proteins via ectodomain interactions [30] . We employed a modified version of the micropatterning assay developed in our laboratory [32] to immobilize and enrich mGFP-GPI in a quantifiable manner within patterned regions directly in the plasma membrane of live cells ( Fig. 1a ). Micropatterning of membrane proteins has been used in several studies to probe functional interactions of patterned proteins with fluorescently labelled interaction partners [33] , [34] . Notably, cells grown on micropatterned antibody against α5β1-integrin showed vascular endothelial growth factor -dependent recruitment of the GPI-anchored protein uPAR to the patterned integrins [35] . To generate functionalized micropatterned surfaces, biotinylated GFP antibody was incubated on coverslips featuring streptavidin patterns produced by microcontact printing. We adjusted the surface density of GFP antibody by adding various concentrations of free biotin to the incubation mix; interspaces were passivated with BSA. Super-resolution microscopy showed that the functional antibody was randomly distributed within the generated patterns ( Fig. 1b ). T24 cells expressing mGFP-GPI were grown on the patterned surfaces, leading to a redistribution and immobilization of the mGFP-GPI in the plasma membrane according to the antibody pattern ( Fig. 1c ). We used these platforms to study the influence of the immobilized mGFP-GPI on the surface distribution and the mobility of different fluorescently labelled probe molecules by comparing data obtained in ‘ON’ versus ‘OFF’ regions of the cells ( Fig. 1d ). We quantified the surface density of immobilized mGFP-GPI via brightness analysis, by referencing the brightness of single GFP molecules (see Methods section). All experiments were performed at mGFP-GPI densities between ρ mGFP-GPI =500 μm −2 and 10,000 μm −2 (ON regions); these densities correspond to characteristic nearest-neighbour distances between d mGFP-GPI =45 and 10 nm. Interspaces had a residual density of immobilized mGFP-GPI of <200 μm −2 (OFF regions). mGFP-GPI areas do not recruit the GPI-anchored protein CD59 In model membranes, Roder et al . [11] found stabilization of ordered phases in micropatterns of tethered saturated lipids. We assumed that, according to the raft hypothesis, it should be possible to induce a similar behaviour in the native plasma membrane: our idea was that micropatterning of mGFP-GPI could nucleate the formation of larger ordered phases in the mGFP-GPI-enriched areas, or at least co-enrich ordered nanosopic phases together with the mGFP-GPI molecules; here and in the following, ‘order’ refers to the lipid acyl chain order. We first evaluated whether the generated mGFP-GPI areas recruited proteins, which are considered to partition into the more ordered raft-like regions of the plasma membranes. The GPI-anchored protein CD59 was consistently found in DRM fractions [36] and was shown to partition into Lo phase regions of GPMVs [37] . We labelled a small fraction of endogenously expressed CD59 via an Atto647N-Fab fragment to record the positions and trajectories of individual CD59 molecules with respect to the pattern geometry. Interestingly, an overlay of all recorded CD59 positions—although not homogeneous in distribution—did not reveal any correlation with the underlying mGFP-GPI pattern ( Fig. 2a ). Quantitative analysis of 31 cells showed no recruitment of CD59 to mGFP-GPI areas, irrespective of mGFP-GPI surface density ( Fig. 2b ). 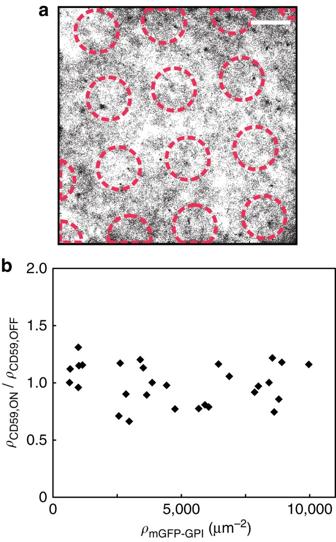Figure 2: CD59 is not recruited to mGFP-GPI areas. (a) The positions of single Fab-Atto 647N-labelled CD59 molecules were recorded within a selected region of interest; no apparent correlation with the underlying mGFP-GPI patterns (red circles) is visible. Scale bar, 3 μm. (b) The relative surface density of CD59,ρCD59,ON/ρCD59,OFF, is plotted as a function of the surface density of mGFP-GPI,ρmGFP-GPI, for 31 individual cells (six independent experiments). Figure 2: CD59 is not recruited to mGFP-GPI areas. ( a ) The positions of single Fab-Atto 647N-labelled CD59 molecules were recorded within a selected region of interest; no apparent correlation with the underlying mGFP-GPI patterns (red circles) is visible. Scale bar, 3 μm. ( b ) The relative surface density of CD59, ρ CD59,ON / ρ CD59,OFF , is plotted as a function of the surface density of mGFP-GPI, ρ mGFP-GPI , for 31 individual cells (six independent experiments). Full size image mGFP-GPI enrichment does not increase the membrane order One characteristic parameter of ordered membranes is the reduced mobility of its constituents compared with the disordered phase ( ∼ 3-fold for GPMVs [38] and ∼ 10-fold for model membranes [39] ). Thus, we were interested whether a probe with equal partitioning between ordered and disordered phases would show differential mobility with respect to the mGFP-GPI patterns. We used Chol-KK114, a cholesterol derivative labelled at the headgroup with the fluorescent dye KK114 via a polyethylene glycol (PEG) linker, which was shown to partition equally between Lo and Ld phases in giant unilamellar vesicles [27] . We further confirmed that it did not show a marked preference for Lo versus Ld regions in GPMVs ( Supplementary Fig. 1 ). The use of a PEG-linker made flip flop of the probe to the inner leaflet of the plasma membrane less likely to occur. As with CD59, we did not observe any correlation of the Chol-KK114 single-molecule positions and the mGFP-GPI pattern ( Supplementary Fig. 2 ). Single-molecule trajectories of Chol-KK114 were recorded and the diffusion coefficients were determined separately for mGFP-GPI-enriched and -depleted areas. 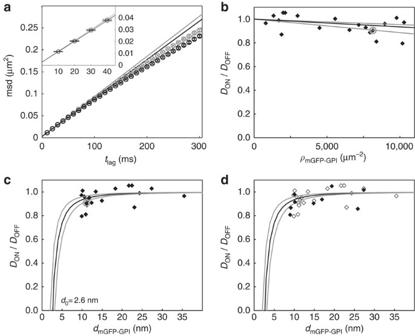Figure 3: Tracer mobility is only minimally affected by mGFP-GPI enrichment. (a) The mean square displacements of Chol-KK114 ON (black) and OFF (grey) mGFP-GPI-enriched areas are plotted as a function oftlagfor one representative cell. Diffusion coefficients were determined by fitting the function MSD=4Dtlag+4σ2xy(bold lines). Only the first two data points were considered for fits. We also included an anomalous diffusion fit with MSD=4Dtlagα+4σ2xy(hairlines), yieldingαON=0.940 andαOFF=0.922. The first 10 data points were considered for fits. The inset shows a magnification of the first four data points. Only minor deviation from Brownian motion was observed ON as well as OFF mGFP-GPI areas. Relative diffusion coefficientsDON/DOFFwere determined for 19 individual cells in four independent experiments and plotted as a function ofbmGFP-GPI densityρmGFP-GPIor (c) average mGFP-GPI spacingdmGFP-GPI. Data were fitted withDON/DOFF=1—d02/dmGFP-GPI2(c) yielding the characteristic nearest-neighbour distance of mGFP-GPI at the percolation thresholdd0=2.6±0.5 nm. The grey circle indicates the ratio of diffusion coefficients shown in (a). The grey lines represent the s.e. of the fit. (d) Relative diffusion coefficientsDON/DOFFof Chol-KK114 as a function of average mGFP-GPI spacingdmGFP-GPIin T24 cells (open diamonds) and in HeLa cells (closed diamonds,N=9, three independent experiments). Figure 3a shows typical curves, in which the mean square displacement (MSD) of Chol-KK114 was plotted against the time lag ( t lag ), both for mGFP-GPI-enriched (ON) and -depleted (OFF) areas. Chol-KK114 showed almost pure Brownian motion in both regions of the pattern and hardly any difference in mobility between ON and OFF areas. Further, the relative diffusion coefficient D ON / D OFF of Chol-KK114 was only slightly reduced (by up to 10%) by the density of immobilized mGFP-GPI ( Fig. 3b ); the effect was too small to be consistent with the formation of a continuous, more ordered membrane phase. Experiments on HeLa cells yielded similar results ( Fig. 3d ). We conclude that no connective ordered phase with raft-like properties was formed by the mGFP-GPI enrichment, even at surface densities of 10,000 mGFP-GPI molecules per μm 2 (corresponding to 10-nm characteristic nearest-neighbour distance), which is already close to the maximum packing density of the GFP. Figure 3: Tracer mobility is only minimally affected by mGFP-GPI enrichment. ( a ) The mean square displacements of Chol-KK114 ON (black) and OFF (grey) mGFP-GPI-enriched areas are plotted as a function of t lag for one representative cell. Diffusion coefficients were determined by fitting the function MSD=4 Dt lag +4σ 2 xy (bold lines). Only the first two data points were considered for fits. We also included an anomalous diffusion fit with MSD=4 Dt lag α +4σ 2 xy (hairlines), yielding α ON =0.940 and α OFF =0.922. The first 10 data points were considered for fits. The inset shows a magnification of the first four data points. Only minor deviation from Brownian motion was observed ON as well as OFF mGFP-GPI areas. Relative diffusion coefficients D ON / D OFF were determined for 19 individual cells in four independent experiments and plotted as a function of b mGFP-GPI density ρ mGFP-GPI or ( c ) average mGFP-GPI spacing d mGFP-GPI . Data were fitted with D ON /D OFF =1 — d 0 2 /d mGFP-GPI 2 ( c ) yielding the characteristic nearest-neighbour distance of mGFP-GPI at the percolation threshold d 0 =2.6±0.5 nm. The grey circle indicates the ratio of diffusion coefficients shown in ( a ). The grey lines represent the s.e. of the fit. ( d ) Relative diffusion coefficients D ON / D OFF of Chol-KK114 as a function of average mGFP-GPI spacing d mGFP-GPI in T24 cells (open diamonds) and in HeLa cells (closed diamonds, N =9, three independent experiments). Full size image Patterned mGFP-GPIs are steric obstacles to probe diffusion We next examined the diffusion behaviour of CD59 with respect to the mGFP-GPI patterns. Moreover, in this case, diffusion in both ON and OFF areas could be well described by free Brownian motion ( Fig. 4a ; diffusion in OFF areas and in cells grown on non-patterned substrates was identical). For CD59, however, mGFP-GPI enrichment had a strong effect on the mobility of the probe: CD59 diffusion was slowed down substantially with increasing mGFP-GPI surface density ( Fig. 4b ). 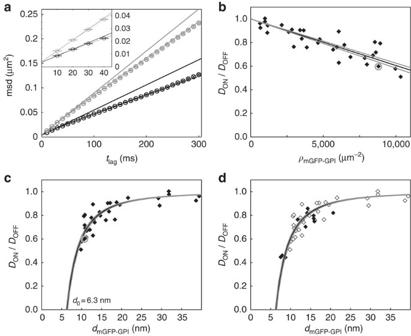Figure 4: Mobility of CD59 decreases linearly with increasing mGFP-GPI surface density. (a) The mean square displacements of CD59 ON (black) and OFF (grey) mGFP-GPI-enriched areas as a function oftlagfor a representative cell. Diffusion coefficients were determined by fitting the function MSD=4Dtlag+4σ2xy(bold lines). Only the first two data points were considered for fits. We also included an anomalous diffusion fit with MSD=4Dtlagα+4σ2xy(hairlines), yieldingαON=0.917 andαOFF=0.949. The first 10 data points were considered for fits. The inset shows a magnification of the first four data points. Relative diffusion coefficientsDON/DOFFof CD59 were determined for 31 individual cells in six independent experiments and plotted as a function of (b) mGFP-GPI densityρmGFP-GPIor (c) average mGFP-GPI spacingdmGFP-GPI. Data were fitted withDON/DOFF=1−d02/dmGFP-GPI2yielding the characteristic nearest-neighbour distance of mGFP-GPI at the percolation thresholdd0=6.3±0.2 nm. The grey circle indicates the data point shown ina. The grey lines represent the s.e. of the fit. (d) Relative diffusion coefficientsDON/DOFFof CD59 as a function of average mGFP-GPI spacingdmGFP-GPIin T24 cells (open diamonds) and in HeLa cells (closed diamonds,N=11, three independent experiments). Figure 4: Mobility of CD59 decreases linearly with increasing mGFP-GPI surface density. ( a ) The mean square displacements of CD59 ON (black) and OFF (grey) mGFP-GPI-enriched areas as a function of t lag for a representative cell. Diffusion coefficients were determined by fitting the function MSD=4 Dt lag +4 σ 2 xy (bold lines). Only the first two data points were considered for fits. We also included an anomalous diffusion fit with MSD=4 Dt lag α +4σ 2 xy (hairlines), yielding α ON =0.917 and α OFF =0.949. The first 10 data points were considered for fits. The inset shows a magnification of the first four data points. Relative diffusion coefficients D ON / D OFF of CD59 were determined for 31 individual cells in six independent experiments and plotted as a function of ( b ) mGFP-GPI density ρ mGFP-GPI or ( c ) average mGFP-GPI spacing d mGFP-GPI . Data were fitted with D ON /D OFF =1− d 0 2 /d mGFP-GPI 2 yielding the characteristic nearest-neighbour distance of mGFP-GPI at the percolation threshold d 0 =6.3±0.2 nm. The grey circle indicates the data point shown in a . The grey lines represent the s.e. of the fit. ( d ) Relative diffusion coefficients D ON / D OFF of CD59 as a function of average mGFP-GPI spacing d mGFP-GPI in T24 cells (open diamonds) and in HeLa cells (closed diamonds, N =11, three independent experiments). Full size image There are two possible reasons for the reduction in CD59 mobility: (i) transient immobilization of CD59 at the immobilized mGFP-GPI tethers, so that the average probe mobility would be a weighted average of mobile and immobile molecules. Probe immobilization, however, would have resulted in its accumulation, which was not observed ( Fig. 2b ); (ii) repulsion of CD59 by impenetrable immobile mGFP-GPI obstacles. The presence of immobile obstacles leads to a linear decrease in the average probe diffusion coefficient with increasing obstacle surface density, which was calculated theoretically [40] and observed experimentally on model membranes [41] . We fitted our data with to yield the characteristic nearest-neighbour distance of obstacles d mGFP-GPI at the percolation threshold, d 0 =6.3±0.2 nm ( N =31; Fig. 4c ). From the fraction of the total area covered by obstacles at the percolation threshold, θ , we can thus estimate the size of obstacles ; in the following we used results by Saxton, who calculated θ for various tracer sizes with respect to the obstacle size, assuming a regular matrix of obstacles [40] . On the basis of X-ray crystallography data, the size of a single GFP molecule was determined to be 3–4 nm (ref. 42 ); the polypeptide chain of CD59 has a size of ∼ 3 nm in the membrane plane [43] , with additional N-oligosaccharides adjacent to the membrane adding 3–6 nm (ref. 44 ). We thus assumed a scenario where the tracer is double the size of the obstacle, which is characterized by θ =0.1559 (ref. 40 ). We calculate an obstacle size of 2.5±0.1 nm and a tracer size of 5.0±0.1 nm, which is in good agreement with the actual dimensions of the exoplasmic domains of mGFP-GPI and CD59. Steric hindrance therefore fully explains the reduced probe mobility in the micropatterned areas. We applied the same fitting model to the Chol-KK114 data, which in fact showed a slight decrease in mobility with increasing mGFP-GPI surface density ( Fig. 3b,c ). In this case, it is not the protein ectodomains but the hydrophobic moieties within the lipid bilayer that largely define the excluded area of obstacle and tracer molecules. The cholesterol molecule itself covers an in-plane area of ∼ 0.25 nm 2 (ref. 45 ), corresponding to a size of ∼ 0.7 × 0.3 nm. In addition, there may be contributions because of the hydrophilic fluorophore KK114. We minimized such contributions by adding a flexible PEG linker to decouple the in-bilayer motion of the cholesterol moiety from the tumbling motion of the fluorophore. The GPI anchor of our mGFP-GPI construct has two to three acyl chains, depending on cell-type-specific efficiency of inositol-deacylation [46] ; a size of ∼ 1.4 × 0.7 nm can be expected. To account for the size difference between cholesterol and the acyl chains of the mGFP-GPI anchor, we assumed twofold smaller tracers than obstacles ( θ ∼ 0.4; ref. 40 ). We thus calculate a tracer size of 0.8±0.2 nm and an obstacle size of 1.6±0.3 nm ( N =19). Therefore, also in this case steric hindrance provides a good quantitative explanation for the reduced cholesterol mobility. Note that incomplete chromophore maturation of mGFP can result in an underestimation of the obstacle density. Considering incomplete maturation of up to 20% (ref. 47 ) our calculation gives slightly smaller reaches of mGFP-GPI of 2.3 nm with respect to CD59, and of 1.5 nm with respect to Chol-KK114. Variations of ρ mGFP-GPI ( ∼ 10% within one pattern) will hardly affect the calculated tracer and obstacle sizes because of the linear relationship of ρ mGFP-GPI and D ON . Effect of cholesterol and temperature Dependence on acute cholesterol depletion has been taken as a hallmark for lipid raft-associated processes. We thus tested whether the observed reduction in CD59 mobility was influenced by cholesterol depletion. The extent of cholesterol depletion by treatment of our cells with cholesterol oxidase (1 U ml −1 ) was determined to be 44% using the Amplex Red cholesterol assay kit. While cholesterol depletion resulted in a slight increase in overall mobility ( Supplementary Table 1 ), it did not have a significant effect on the relative diffusion coefficients D ON/OFF ( Fig. 5a ). 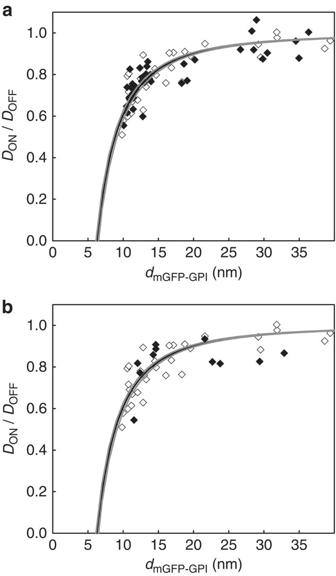Figure 5: Effect of cholesterol depletion and temperature change on CD59 mobility. (a) Relative diffusion coefficientsDON/DOFFof CD59 as a function of average mGFP-GPI spacingdmGFP-GPI(open diamonds) and after treatment with 1 U ml−1cholesterol oxidase (closed diamonds;N=34, six independent experiments). (b) Relative diffusion coefficientsDON/DOFFof CD59 as a function of average mGFP-GPI spacingdmGFP-GPIat 23 °C (open diamonds) and at 37 °C (closed diamonds;N=11, three independent experiments). Figure 5: Effect of cholesterol depletion and temperature change on CD59 mobility. ( a ) Relative diffusion coefficients D ON / D OFF of CD59 as a function of average mGFP-GPI spacing d mGFP-GPI (open diamonds) and after treatment with 1 U ml −1 cholesterol oxidase (closed diamonds; N =34, six independent experiments). ( b ) Relative diffusion coefficients D ON / D OFF of CD59 as a function of average mGFP-GPI spacing d mGFP-GPI at 23 °C (open diamonds) and at 37 °C (closed diamonds; N =11, three independent experiments). Full size image Finally, also temperature has a pronounced effect on membrane fluidity and is known to influence phase separation, for example, in GPMVs [37] . We therefore repeated our experiments at 37 °C: the overall diffusion coefficients of CD59 were increased ( Supplementary Table 1 ); still, the dependence of D ON / D OFF on d mGFP-GPI was not changed compared with data recorded at room temperature ( Fig. 5b ). Neither cholesterol depletion nor temperature increase did alter the distribution of CD59 with respect to mGFP-GPI patterns ( Supplementary Fig. 3 ). In this study we show that immobilized mGFP-GPI molecules can be viewed as independent obstacles to the diffusion of other membrane constituents; particularly, they do not act collectively by nucleating the formation of connective-ordered regions in the plasma membrane. From our results we inferred the distance over which single immobilized GPI-anchored proteins influence their environment in the native plasma membrane. We found this reach to be determined essentially by the size and the shape of the mGFP-GPI: the GFP moiety of ∼ 2.5 nm diameter limits the approach of membrane constituents, which protrude into the extracellular space; the acyl chains of the GPI anchor set the ultimate limit of ∼ 1.6 nm for the approach of lipids, which can huddle underneath the protein ectodomain. On the basis of our data we can further rule out the presence of substantial attractive ‘raft-type’ forces transiently recruiting and trapping other raft markers. In the following we discuss implications of our findings. First, we find that local enrichment of Lo phase markers does not nucleate the formation of ordered membrane phases. Lo and Ld phase markers are segregated into distinct regions of phase-separated membranes, depending on their particular partition coefficient. In turn, clustering and pinning of Lo phase markers nucleates the formation of ordered membrane regions or recruits pre-existing ordered nanodomains, as proposed in Ehrig et al . [20] and Machta et al . [19] , and observed in model membrane systems [11] , [12] . We did not find according effects in the plasma membrane of live cells; instead our results are in line with previous data, where no evidence for nanodomains based on lipid-mediated phase separation [48] or co-diffusion of different GPI-anchored proteins have been found [30] , [49] . In the following, we provide arguments why the currently discussed models of membrane rafts are incompatible with our data. Estimates of the plasma membrane area fraction constituted by an ordered lipid phase, f Lo , range from 10 to 44%, depending on temperature, cell type and method used [26] , [50] , [51] , [52] . In our assay, mGFP-GPI-enriched regions cover an area fraction f GPI ∼ 16% of the cell membrane. In those ON regions, one would have expected the formation of a continuous ordered phase: the density of GPI-APs is increased up to a hundredfold compared with an untreated cell [53] , and the characteristic nearest-neighbour distances are well below the expected correlation length of critical fluctuations in GPMVs of ∼ 20 nm (ref. 19 ). If we assume here that the overall lipid composition is not affected by our micropatterning assay, we may expect that also the OFF regions contain a residual proportion of ordered phase of , yielding 0–33%. This is, however, not what we observed: first, we did not find the concomitant enrichment of CD59 in the ON regions. At least threefold enrichment would have been expected, considering CD59’s >90% Lo phase partitioning [37] . Second, we did not detect a substantial decrease in Chol-KK114 mobility in ON regions. The diffusion constant of Chol-KK114 should have been affected according to ; with f Lo , OFF =0–33% and (ref. 38 ), a 2.34- to 3-fold reduction in mobility ON versus OFF would have been expected. The more recent literature turned ambiguous about the amount of ordered versus disordered phase that can be expected in the plasma membrane. Some studies indicate much higher fractions of ordered phase than previously assumed [22] , [38] ; for example, Owen et al . [22] calculated f Lo =76% ordered phase in HeLa cells, which was reduced to 30% on cholesterol extraction. Even if we take the data reported in ref. 22 ., we would have expected a 1.4-fold enrichment of CD59 in the ON regions and a 1.6-fold reduction in Chol-KK114 mobility in ON versus OFF regions, which was not detected. Further, cholesterol depletion should have massively reduced the residual ordered phase in the OFF regions ( f Lo,OFF ∼ 16%, assuming f Lo =30%), resulting in a substantial increase in CD59 enrichment (approximately sixfold) and Chol-KK114 retardation (2.7-fold), which was also not observed. We interpret this discrepancy in view of annular lipids, which, because of their tight association with membrane proteins, may have completely different properties such as altered rotational and translational mobility as well as acyl chain order [4] . These annular lipids are expected to constitute a substantial fraction of lipids in the plasma membrane [4] , [5] . Overall, it seems that the outer leaflet of the plasma membrane is in a uniform lipid phase state, and does not show Lo/Ld phase coexistence. This finding contrasts with observations from synthetic lipid mixtures and GPMVs, where large-scale phase separation has frequently been observed. However, increasing the complexity of a lipid mixture also increases the maximum amount of phases that may coexist; in a cell membrane we may expect thousands of different lipid species, and consequently up to thousands of coexisting lipid phases. Experimentally, this plethora of phases would be difficult to discriminate. It was thus surprising to see that GPMVs resemble the characteristics of much simpler ternary lipid systems by showing Lo/Ld phase separation and domain fluctuations reminiscent of critical behaviour [18] . When trying to understand the differential behaviour of lipids in GPMVs versus the cellular plasma membrane, we have to consider the main differences between the two systems. First, the anisotropic lipid composition between the two membrane leaflets is lost in GPMVs. Both head group charge and the degree of acyl chain saturation are substantially different in the inner and outer leaflets of the plasma membrane [54] ; therefore, the mixing of inner and outer leaflet lipids may well facilitate the observed phase separation. Second, GPMVs are devoid of the actin membrane skeleton. In the plasma membrane, a large fraction of proteins—and thus of the bound annular lipids—is immobilized via the actin skeleton; those molecules do not participate in the equilibration of the live cell system, but they do equilibrate in GPMVs. Third, nearly all model membranes and GPMVs were studied at zero membrane tension. The actin skeleton, however, imposes tension on the natural plasma membrane, which introduces an additional degree of freedom, with a priori unknown consequences on the phase coexistence behaviour. In conclusion, our results corroborate a scenario where phase partitioning is not a fundamental element of protein organization and mobility in the live cell plasma membrane. This further implies that, in a live cell, lipid phase separation does not provide the means of modulating protein localization and interactions as the raft hypothesis would suggest. Our second major finding is that GPI-anchored proteins per se do not represent interaction sites for other proteins. There are frequent reports in the literature that GPI-anchored proteins do not diffuse randomly in the plasma membrane, but instead show frequent halts in a cholesterol-dependent manner [28] , [55] . Partitioning into pre-existing lipid–protein complexes, their de novo assembly, or lipid shells [56] were proposed as possible models. More recently, however, the Kusumi laboratory has found that for GPI-anchored proteins it is the protein ectodomains—and not the GPI-anchor itself—which dominate the interaction between GPI-anchored proteins [30] . Consistent with the results presented in ref. 30 , our data allow for ruling out specific transient halts of CD59 at the immobilized mGFP-GPI molecules (a direct comparison of our findings with those of ref. 30 can be found in Supplementary Note 1 ). Let us assume that such transient association indeed occurred, and that the tracers spent on average a proportion β of their time in the freely diffusing state; as a quantitative example, β ∼ 65% was measured in ref. 28 . The consequence would have been an enrichment of tracers according to ρ ON / ρ OFF = β −1 ∼ 1.5, which was not observed in our study ( Supplementary Fig. 4 ). The same holds true for the Chol-KK114; also in this case, the absence of probe enrichment in the mGFP-GPI micropatterns ( Supplementary Fig. 2 ) allows for excluding transient deceleration at the immobilized mGFP-GPI molecules. This provides an additional argument against the presence of nanoscopic ordered domains associated with GPI-anchored proteins. In a recent publication it was suggested that most membrane proteins are assembled in mesoscale domains at the plasma membrane, and that diffusion within those assemblies is significantly slowed down [27] . Further, a moderate but significant enrichment of a model GPI-AP within multiprotein assemblies was reported. Our experiments indicate that the reverse is not true: immobilization and enrichment of mGFP-GPI does not trigger recruitment of CD59 ( Fig. 2 ); in addition, also unspecific recruitment of membrane proteins to mGFP-GPI areas can be ruled out as this would have reduced the mobility of Chol-KK114 in ON regions and increased the determined size of the mGFP-GPI obstacles by the size of the recruited proteins. Finally, we find that immobilized mGFP-GPIs essentially behave as inert obstacles that reduce the mobility of other membrane constituents according to their molecular size and shape. There has been a long-lasting debate on the question, why diffusion in the plasma membrane is much slower than in model membranes. Recent discussion has focused on the lipid bilayer itself: the retardation was attributed, for example, to periodic barriers, which separate compartments of high fluidity [57] , but also partitioning to lipid domains of higher order and lower fluidity was proposed [22] . The diffusion constant of a given membrane protein, however, depends not only on the frictional coefficient in the bilayer region itself ( f b ), but also in membrane-proximal exoplasmic ( f e ) and cytoplasmic layers ( f c ), which add linearly to the total friction according to D = kT /( f e + f b + f c ) (ref. 58 ). Both cytoplasmic [57] , [58] and exoplasmic layers [59] , [60] were observed to influence protein mobility. Indeed, the immediate environment of the plasma membrane is densely packed with proteins protruding into the exoplasmic and cytoplasmic space [61] . The packing density depends on the distance z from the membrane surface: while the transmembrane regions may actually be wider-spaced, exoplasmic domains contain bulky polypeptide chains and glycosylations, and cytoplasmic domains are frequently decorated with adapter proteins and other signalling molecules. Depending on its shape, a moving molecule in the membrane will thus frequently experience void areas, which propel the random walk of the tracer. The process is similar to the free area model proposed for lipid diffusion [62] . Immobilized, but also high concentrations of mobile obstacles lead to a retardation of diffusing tracers [63] . To account for differences of friction along the membrane normal, we can assume different degrees of crowding, which are experienced by tracer A at different distances from the membrane surface. For this, we introduce a differential frictional coefficient . If we neglect hydrodynamic interactions between individual layers, the tracer diffusion constant is given by . In other words, as we move away from the surface along the membrane normal, each segment of a tracer, d z , senses a characteristic friction, f A ( z ), as sketched in Fig. 6 . The reach of a membrane-associated molecule A with respect to a second molecule B can be defined as its repulsion diameter δ A->B . In this work, we have determined a repulsion diameter of mGFP-GPI with respect to CD59 of 2.5 nm, which agrees well with the diameter of the GFP β-barrel of 3 nm. The reach of mGFP-GPI with respect to the cholesterol analogue Chol-KK114 is much shorter: the lipid is not hindered by the mGFP ectodomain and thus experiences a smaller obstacle size of 1.6 nm, close to the actual size of the GPI-anchor’s acyl chains. It should be noted that mGFP-GPI dimers [31] would most likely not be detectable by this approach. 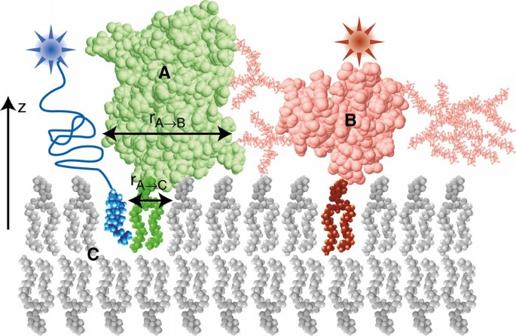Figure 6: Tracers experience varying degrees of friction at different distances from the membrane surface. The reach of a membrane-associated moleculeAwith respect to a second moleculeBcan be defined as its repulsion diameterδA→B. For the interaction pair mGFP-GPI (green) and CD59 (red),δmGFP-GPI→CD59is determined by the GFP moiety and the glycosylated exoplasmic part of CD59 yieldingδmGFP-GPI→CD59=2.5 nm. In contrast, Chol-KK114 (blue) can approach the acyl chains of the GPI anchor, giving rise to a repulsion diameterδmGFP-GPI→Chol-KK114of 1.6 nm. Figure 6: Tracers experience varying degrees of friction at different distances from the membrane surface. The reach of a membrane-associated molecule A with respect to a second molecule B can be defined as its repulsion diameter δ A→B . For the interaction pair mGFP-GPI (green) and CD59 (red), δ mGFP-GPI→CD59 is determined by the GFP moiety and the glycosylated exoplasmic part of CD59 yielding δ mGFP-GPI→CD59 =2.5 nm. In contrast, Chol-KK114 (blue) can approach the acyl chains of the GPI anchor, giving rise to a repulsion diameter δ mGFP-GPI→Chol-KK114 of 1.6 nm. Full size image In conclusion, our data show that GPI-APs do not influence their membrane environment over distances beyond their actual physical size by stabilizing ordered membrane domains. Instead, the reach of a GPI-AP in the native plasma membrane is determined essentially by its molecular size and shape. In this context it is interesting to note that steric factors were indeed observed to affect the uptake of membrane molecules via clathrin-mediated endocytosis [64] : GPI-anchored proteins and synthetic lipid-anchored proteins were excluded from the rather crowded environments of clathrin-coated pits because of their bulky ectodomains, while membrane lipids were not. DNA and reagents The pCR3 mGFP-GPI(DAF (decay-accelerating factor)), a GFP modified by the GPI anchor of DAF (CD55/DAF), was kindly provided by Daniel Legler (University of Konstanz, Switzerland). The GFP of this vector was mutated at amino-acid position 206 from alanine to lysine to get a mGFP variant [65] . The monoclonal biotinylated antibodiy against GFP (clone 9F9.F9) was purchased from Novus Biologicals, CO. The Atto647N-labelled Fab fragment against CD59 and the HeLa cell line were a gift from H. Stockinger (Medical University of Vienna, Austria). Cholesterol oxidase from Streptomyces sp. was purchased from Sigma-Aldrich. Chol-KK114 was kindly provided by V. Belov (Max-Planck Institute for Biophysical Chemistry, Göttingen, Germany). Micropattern production Microstructured surfaces were made following a protocol adapted from ref. 32 . Briefly, polydimethylsiloxane (PDMS) stamps bearing circular features with a diameter of 3 μm and a distance of 3 μm were incubated with 50 μg ml −1 streptavidin in PBS for 15 min, rinsed with PBS and dH 2 O and dried with N 2 . Immediately after drying, the stamp was placed on an epoxy-coated coverslip (Schott) and incubated for 30 min at room temperature. After removal of the stamp, the coverslip was incubated with biotinylated GFP antibody at a concentration of 10 μg ml −1 in PBS with 1% BSA. For some samples, biotin (5–50 ng ml −1 ) was included in the antibody mixture to adjust lower densities of bound antibody and consequently lower densities of immobilized mGFP-GPI. Cell culture The human bladder carcinoma cell line T24 (DSMZ no. ACC 310, Leibniz Institute DSMZ) stably transfected with mGFP-GPI(DAF) was cultured in RPMI 1640 medium containing 10% fetal calf serum (FCS). HeLa cells were cultured in Dulbecco’s Modified Eagle Medium/HAMS F-12 Medium 1/1 supplemented with 2 mM L-glutamine and 10% FCS. Cells were grown in a humidified atmosphere at 37 ° C and 5% CO 2 . HeLa cells were transiently transfected with mGFP-GPI(hFR) using the TurboFect Transfection Reagent (Thermo Scientific) 24 h before experiments according to the manufacturer’s protocol. For micropatterning experiments, cells were grown to 80% confluency and harvested by treatment with accutase. Cells were seeded on the micropatterned surfaces in Secure-Seal hybridization chambers (Grace Biolabs) and grown for 2 h before measurements. For cholesterol depletion, patterned cells were incubated in the presence of 1 U ml −1 cholesterol oxidase in HBSS at 37 °C for 20 min. The extent of cholesterol depletion was determined using the Amplex Red Cholesterol Assay Kit (Invitrogen) following the manufacturer’s instructions. GPMV preparation and microscopy GPMVs were obtained as described in ref. 66 . Briefly, cells grown to 80% confluency were washed twice with PBS and blebbing was initiated by adding a buffer composed of 2 mM CaCl 2 , 10 mM Hepes and 0.15 M NaCl at pH 7.4, to which formaldehyde and dithiothreitol at final concentrations of 25 and 2 mM, respectively, were added. After 2 h of incubation at 37 °C GPMVs that had separated from the cell monolayer were gently decanted into a 15-ml conical tube and stored at 4 °C to settle. GPMVs were stained with the Ld marker DiI (2 μg ml −1 ) and Chol-KK114 (0.5 μg ml −1 ) and imaged on a Zeiss LSM700 confocal microscope at 10 °C. The partitioning of Chol-KK114 into Lo and Ld phases was quantified as described in ref. 66 using the Zeiss’ ZEN software. Briefly, the Ld phase was identified by the presence of the DiI marker and the partitioning of Chol-KK114 was quantified by a fluorescence intensity line scan through the two phases. The Ld partition coefficient %Ld is given by , with F Ld and F Lo being the background-corrected fluorescence intensities of Chol-KK114 in the Ld and Lo phases, respectively. Total internal reflection fluorescence microscopy Total internal reflection fluorescence microscopy experiments were performed on a home-built system based on a Zeiss Axiovert 200 microscope equipped with a 100 × numeric aperture=1.46 Plan-Apochromat objective (Zeiss). Samples were illuminated stroboscopically using a 488-nm OPSL laser (Coherent) for excitation of mGFP-GPI, or a 642-nm diode laser (TOPTICA) for excitation of the Atto647N-Fab or Cholesterol-KK114. After appropriate filtering, the fluorescence signal was recorded on an Andor IXON Ultra EMCCD camera. Determination of mGFP-GPI density and distribution All cell measurements were carried out in HBSS supplemented with 2% FCS at 23 °C unless indicated otherwise. The mGFP-GPI density ρ mGFP-GPI specifies the number of mGFP-GPI molecules per μm 2 ; it was determined by relating the mean bulk brightness of the mGFP-GPI-enriched (ON) areas with the brightness of single mGFP-GPI molecules. For determination of the single molecule brightness, we performed a variant of our TOCCSL method [31] on cells seeded on unpatterned regions of the glass slide. Briefly, a rectangular region of interest was completely photobleached by a strong laser pulse. After a recovery time of 5 s, we recorded sequences of 30 images, which contained well-separated signals of single or dimeric mGFP-GPI molecules. For determination of the single molecule brightness we discarded the first 10 images to avoid detection of mGFP-GPI dimers. This was repeated several times. Single molecules were identified and their brightness analysed using in-house algorithms implemented in MATLAB (MathWorks) [31] . The median of the intensity values was taken for the single mGFP brightness. We determined the number of immobilized mGFP-GPIs for every region, where single-molecule diffusion was measured. The mean pixel intensity values of OFF area regions were subtracted from the mean pixel intensity values of ON regions to determine the intensity contribution of immobilized mGFP-GPI species. The resulting mean pixel intensity of immobilized mGFP-GPI was divided by the single-molecule brightness to yield the surface density ρ mGFP-GPI . The characteristic centre–centre distance is given by . Distribution of functional antibody was monitored via photoactivated localization microscopy (PALM) experiments. For this, we bound soluble psCFP2 (1 μM in PBS +1% BSA) to the micropatterned GFP antibody, which also recognizes psCFP-2. Light (488 nm) was used both for photoactivation and imaging of psCFP-2. A series of 10,000 PALM images was taken with illumination times of 5 ms. Recorded images were analysed using algorithms implemented in MATLAB as described in ref. 67 . The data were corrected for localizations of the same molecule in consecutive images. Chol-KK114 and CD59 distribution and diffusion Micropatterned cells were incubated with either Chol-KK114 (20 ng ml −1 ) or anti-CD59 Fab-Atto647N (50 pM) in HBSS containing 2% FCS for 10 min and washed. After taking an mGFP-GPI pattern image, movies of Chol-KK114 or CD59 were recorded at an illumination time of 3 ms and a frame rate of 10 ms. Images were analysed using in-house algorithms implemented in MATLAB [68] . To determine probe diffusion coefficients respective to the mGFP-GPI pattern, trajectories were divided into the two fractions ON and OFF using selection masks made from the underlying mGFP-GPI images. The MSDs were plotted against the time lag and the diffusion coefficient was determined by fitting the function MSD=4 Dt lag +4 σ 2 xy , where σ xy denotes the localization precision (for CD59-FabAtto647N we found σ xy =30±1 nm, for Chol-KK114 σ xy =27±1 nm); diffusion coefficients were determined from the first two data points. To determine the apparent anomalous diffusion coefficient and the anomalous exponent α we used the function MSD=4 D α t lag α +4 σ 2 xy . From the probe diffusion coefficients D ON and D OFF , we calculated the relative diffusion coefficient D ON / D OFF and plotted it against mGFP-GPI surface density ρ mGFP-GPI and characteristic distance d mGFP-GPI . The mobility of a diffusing particle decreases linearly with obstacle surface density down to the percolation threshold, where D ON / D OFF =0 (ref. 40 ). Thus, we fitted our data with D ON /D OFF =1— d 0 2 /d mGFP-GPI 2 to yield the characteristic nearest-neighbour distance d 0 at the percolation threshold. The fraction of the total area covered by obstacles at the percolation threshold, θ , depends on the size of obstacle and diffusing particle [40] ; on the basis of the relative molecular sizes of obstacle and tracers we assumed θ =0.1559 for CD59 (tracer twice the size of obstacle) and θ ∼ 0.4 for Chol-KK114 (obstacle twice the size of tracer) [40] and calculated the obstacle size (diameter) . How to cite this article: Sevcsik, E. et al . GPI-anchored proteins do not reside in ordered domains in the live cell plasma membrane. Nat. Commun. 6:6969 doi: 10.1038/ncomms7969 (2015).